Trapping red blood cells in living animals using optical tweezers The recent development of non-invasive imaging techniques has enabled the visualization of molecular events underlying cellular processes in live cells. Although microscopic objects can be readily manipulated at the cellular level, additional physiological insight is likely to be gained by manipulation of cells in vivo , which has not been achieved so far. Here we use infrared optical tweezers to trap and manipulate red blood cells within subdermal capillaries in living mice. We realize a non-contact micro-operation that results in the clearing of a blocked microvessel. Furthermore, we estimate the optical trap stiffness in the capillary. Our work expands the application of optical tweezers to the study of live cell dynamics in animals. The biological research in vitro may not reflect the biological activities in vivo accurately because of the complexity of the in vivo environment. Therefore, biological studies in vivo , especially in living animals, are important to verify our knowledge acquired from the in vitro studies. The studies of in vivo biological activities will be greatly accelerated by a tool that allows trapping and manipulation of biological cells within living animals. Although some manipulation techniques for microscopic particles in vitro exist, including optical tweezers [1] , [2] , atomic force microscopy [3] , magnetic tweezers [4] and biomembrane force probe [5] , trapping and manipulation of cells within a living animal has not been reported to the best of our knowledge. Atomic force microscopy and biomembrane force probe can trap and manipulate the cells with mechanical contact force. Magnetic tweezers can manipulate magnetic beads, which are attached to the tethering surface by molecule chain. However, it cannot trap the cells without the help of tethering chain. Those techniques, except for optical tweezers, cannot trap and manipulate the cells within living animals non-invasively because of the limitation of their operating principle. Optical tweezers (originally called ‘single-beam gradient force trap’) [1] , [2] are capable of trapping microscopic particles in vitro [6] , [7] , [8] , [9] or organelles within cells [10] , [11] , [12] , [13] with non-contact force by photon linear momentum transfer. They have been widely used in applications ranging from particle sorting [6] , [7] , [8] to microfabrication [14] , [15] , [16] . Moreover, optical tweezers can be used as a quantitative tool on biophysical research, for example, measuring single molecule binding force [17] , studying kinetochore–microtubule interaction [18] and quantifying intercellular interactions [19] . Optical tweezers have the advantage to actualize the trapping and manipulation of the biological cells within living animals non-invasively, as the laser is able to penetrate through biological tissues. Here we demonstrate how to trap and manipulate the red blood cells (RBCs) within living mice in three dimensions, using optical tweezers. We also quantify the optical stiffness on the cells and show that blood flow in the capillary can be recovered with the help of optical tweezers. Optical trapping and manipulation of RBCs in vivo The depth of blood capillaries in the ear of a mouse is close to the working distance of the optical tweezers. Generally, RBCs in capillaries flow at a speed of 0.1~2 mm s −1 . When the blood flow slows down to a certain degree, RBCs are trapped and held in the optical trap. For a capillary with ~5 μm diameter observed at the depth of ~40 μm beneath the surface of mouse ear skin, the RBCs can only flow one by one in the capillary. The optical trapping of RBCs in the capillary is a gradual process as shown in Fig. 1 and Supplementary Movie S1 . The laser power is estimated to be 168 mW at the trapping location. The RBCs flow through the capillary quickly at the beginning. When the optical trap is located at the centre of the capillary, the speed of RBCs slows down due to attractive action of optical trap. Those RBCs further slow down the blood flow, because the RBCs are about as large as the capillary. The drag force on the RBCs by the flow diminishes gradually due to the slowdown of blood flow. The RBCs can be trapped when trapping force overcomes the drag force. 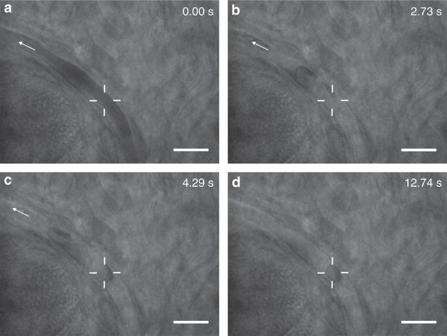Figure 1: Optical trapping of a single RBC. (a) When initiating the optical trap, blood flow is so fast that a single cell cannot be distinguished. (b) The flow then slows down gradually so that single RBC can be distinguished upon optical tweezers. (c) After 4.29 s, optical tweezers trap a RBC whereas other RBCs are still flowing past. (d) The cell is held in the trap, and other RBCs flow out of the view. See alsoSupplementary Movie S1. Scale bar, 10 μm. ‘+’ indicates the optical trap center and arrows indicate the direction of blood flow. Figure 1: Optical trapping of a single RBC. ( a ) When initiating the optical trap, blood flow is so fast that a single cell cannot be distinguished. ( b ) The flow then slows down gradually so that single RBC can be distinguished upon optical tweezers. ( c ) After 4.29 s, optical tweezers trap a RBC whereas other RBCs are still flowing past. ( d ) The cell is held in the trap, and other RBCs flow out of the view. See also Supplementary Movie S1 . Scale bar, 10 μm. ‘+’ indicates the optical trap center and arrows indicate the direction of blood flow. Full size image When the capillary is about as large as the RBCs, the capillary wall is helpful to hold the RBCs. The friction between the capillary wall and trapped cell will hinder the trapped cell to escape from the trap. In the longitudinal direction, the capillary wall can hold up the cell to avoid the longitudinal escaping. The RBCs flow faster in large blood vessel; therefore, higher laser power is required for sufficient transverse gradient force to trap the cells. We increase the laser power and trap an RBC in a vessel with a diameter of ~16 μm at the depth of 45 μm, as shown in Fig. 2 and Supplementary Movie S2 . We manipulate the cell transversally with a passive manipulation method, in which the laser beam is stationary, whereas we move the stage to move the mouse ear. As the sample stage moves transversely, the trapped cell is gradually getting close to the edge of blood vessel as shown in Fig. 2a . The longitudinal manipulation of trapped cell is implemented with active manipulation method, in which the optical trap is moving with the movement of the microscope objective. In Supplementary Movie S2 , the cell moves ~6 μm from the initial trapped site to the final position. The process of longitudinal manipulation is shown in Fig. 2c . When the objective is moving longitudinally, the trapped cell is always in focus while the image of the surrounding tissue becomes blurred, because the surrounding tissue is gradually out of focus. Our results show that optical tweezers can be a useful tool for manipulation of cells in three dimensions within living mice. In the experiments, we also observe that other cells in addition to RBCs can be trapped by optical tweezers, as shown in Supplementary Movie S3 . The cell in Supplementary Movie S3 has a different shape compared with RBCs, and could be an immune cell. 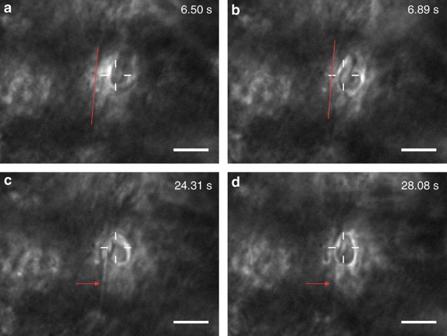Figure 2: Optical manipulation of a RBC in three dimensions. (a,b) Transversal manipulation of a RBCs. The red line indicates the edge of the vessel. The cell moves with a transversal distance of about 4 μm. (c,d) Longitudinal manipulation of a RBCs. The red arrow indicates the edge of the vessel. With the longitudinal movement of the optical trap, the clear image (c) of the vessel edge becomes blurred (d), whereas the trapped RBC image is always clear, indicating that the trapped RBC is moving longitudinally with the optical trap. See alsoSupplementary Movie S2. Scale bar, 10 μm; ‘+’ indicates the optical trap centre. Figure 2: Optical manipulation of a RBC in three dimensions. ( a , b ) Transversal manipulation of a RBCs. The red line indicates the edge of the vessel. The cell moves with a transversal distance of about 4 μm. ( c , d ) Longitudinal manipulation of a RBCs. The red arrow indicates the edge of the vessel. With the longitudinal movement of the optical trap, the clear image ( c ) of the vessel edge becomes blurred ( d ), whereas the trapped RBC image is always clear, indicating that the trapped RBC is moving longitudinally with the optical trap. See also Supplementary Movie S2 . Scale bar, 10 μm; ‘+’ indicates the optical trap centre. Full size image Blockage of the capillary Optical tweezers can induce artificial clot of RBCs in capillaries. For the capillary in Fig. 1 , the diameter of RBC is approximately equal to the capillary diameter. Therefore, one trapped RBC can block the capillary. The trapped RBC causes the artificial clot and finally blocks the blood flow in the capillary as shown in Fig. 1d . The flood flow diverts to other interlinked capillaries, whereas we observe that no other RBCs flow through the capillary within 1 min. For the capillary with a larger diameter than RBCs, optical tweezers can trap a number of RBCs and induce artificial clot as shown in Fig. 3 and Supplementary Movie S4 . The trapping of RBCs leads to the occupation of more free-flow area of the capillary by the trapped RBCs, which ultimately leads to aggregation and capillary blockage. 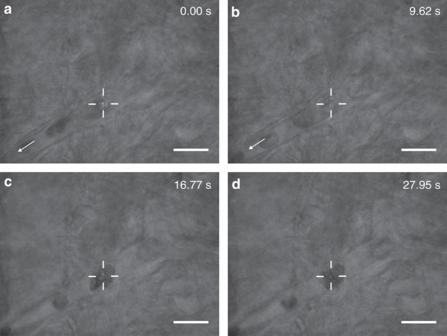Figure 3: Optical trapping of a number of RBCs leads to capillary blockage. (a) Initially, the blood flows quickly through the capillary. (b) Blood flow slows down when optical tweezers trap a cell. However, the capillary is not completely blocked. (c,d) More and more RBCs are trapped, until the blood capillary is blocked completely. See alsoSupplementary Movie S4. Scale bar, 10 μm; ‘+’ indicates the optical trap centre and arrows indicate the direction of blood flow. Figure 3: Optical trapping of a number of RBCs leads to capillary blockage. ( a ) Initially, the blood flows quickly through the capillary. ( b ) Blood flow slows down when optical tweezers trap a cell. However, the capillary is not completely blocked. ( c , d ) More and more RBCs are trapped, until the blood capillary is blocked completely. See also Supplementary Movie S4 . Scale bar, 10 μm; ‘+’ indicates the optical trap centre and arrows indicate the direction of blood flow. Full size image Micro-operation to clear a blocked capillary When a blood capillary is blocked by trapped RBCs, the blood flow is diverted to other capillaries. The cells in the upper direction opposite to the blood flow stop flowing due to the balance of blood pressure. Then, a tube with no flow is sealed by trapped cells and the cells in the upper direction opposite to the blood flow. After a long time, the sealed tube becomes stable and the blood flow is blocked, even when the optical tweezers are turned off. The RBC serves a vital role as an oxygen carrier. Aggregation of RBCs is a very important and vital biological process, which influences the rheological properties of blood and may lead to severe vascular problems. The recovery of the blood flow by an external tool is a useful micro-operation. Here such micro-operation is demonstrated by removing the blockage with optical tweezers. In Fig. 4 and Supplementary Movie S5 , optical tweezers trap the RBCs, which have blocked the capillary, and remove them from the capillary. We slowly apply force to the cell and stop after observing a slight displacement. If the cell is out of the trap centre, we wait for the cell trapping to occur. Therefore, it is possible to advance step by step with increasing displacements, until large changes are made at the position of the cell. With the advancing of the trapped cell, the sealed tube is becoming longer and pressure balance on the cells in the upper direction opposite to the blood flow is changed gradually. Those cells in the upper direction opposite to the blood flow move under the blood pressure from the heart beating; therefore, the capillary is filled with new blood. When the drag force overcomes the friction, the blood flow will flush the blockage after optical tweezers are turned off. At last, the blood flow is recovered in the capillary. The clearance of blocked capillary takes ~35 s in Supplementary Movie S5 . This demonstration shows that optical tweezers might be useful in the treatment of thrombosis. 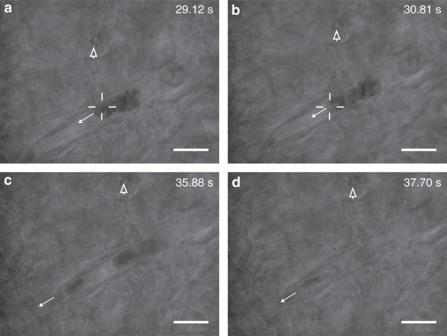Figure 4: Optical tweezers clear a clogged capillary. (a,b) Trapped RBCs move along the capillary with optical trap moving. The RBC remains in the optical trap during movement. (c) The moving distance of the RBC is about 12 μm. The other stationary RBCs in blood capillary start to move when the optical tweezers are turned off. (d) The blood flow returns to normal flow. See alsoSupplementary Movie S5. Scale bar, 10 μm; ‘+’ indicates the optical trap centre and arrows indicate the direction of blood flow, whereas the hollow arrows mark the location of the same surroundings. Figure 4: Optical tweezers clear a clogged capillary. ( a , b ) Trapped RBCs move along the capillary with optical trap moving. The RBC remains in the optical trap during movement. ( c ) The moving distance of the RBC is about 12 μm. The other stationary RBCs in blood capillary start to move when the optical tweezers are turned off. ( d ) The blood flow returns to normal flow. See also Supplementary Movie S5 . Scale bar, 10 μm; ‘+’ indicates the optical trap centre and arrows indicate the direction of blood flow, whereas the hollow arrows mark the location of the same surroundings. Full size image Optical trap stiffness in vivo Biomolecular interactions can generate tiny forces in the pico-Newton range. In the last two decades, optical tweezers has been used to quantify such forces that contribute to cellular and molecular systems. The calibration of optical trap stiffness k is the basis of force measurement. However, because of the complexity of in vivo situation, the methods [20] , such as viscous drag method or power spectrum method, cannot be used to calibrate optical trap stiffness in vivo . Here we attempt to determine optical trap stiffness in vivo with dynamic viscous drag force method [21] . We define x as the distance between the cell centre and the laser focal point. The cell is mainly exerted by the trapping force and the drag force from blood plasma during the motion in the potential well. When the RBC arrives at the edge of the well with a certain velocity, it is attracted by the optical force and accelerated to reach the trap centre. Then the cell is decelerated before it arrives at the maximum deviation displacement ( x = x max ). After the cell reaches the position of x max , the cell gradually backs to the trap centre due to the attractive action of optical force. Here we ignore the slight difference between the trap centre and the final stabilized position caused by low capillary blood pressure at the moment of blocking. We then analyse cell movement trajectory (from x max to the trap centre) to calibrate the optical stiffness. The dynamics equation for the motion of the cell with mass m is when the radius of the cell is close to the radius of the capillary, the most significant factor for the drag force is the ratio of cell radius to capillary radius. The influence of cell shape on the drag force is minor [22] . Then, here the cell in the capillary can be simplified as a rigid sphere with radius a , which is moving along the centreline of a cylindrical tube with radius R . The drag force on a sphere in motion within a moving liquid is composed of two parts: (1) the drag due to the motion of the sphere with velocity U in a still liquid and (2) the drag to the sphere held fixed within a moving liquid having a parabolic velocity distribution (maximum velocity V ). The drag force can be written as [23] where μ is the viscosity of the blood plasma, about 1.2 × 10 −3 Pa s at 37 °C [22] , K 1 and K 2 are functions of a / R and wall correction factors, which weight the contributions from the particle and fluid velocities, respectively. When the RBC is moving in the capillary, the Reynolds number is less than 10 −2 ; therefore, the effect of inertia force can be ignored [24] . Then equation 1 can be written as here we assume that V is a constant during the process of backing to trap centre from x max . Then the solution for equation 3 is an exponential form: . The values of K 1 and K 2 in Supplementary Movie S1 are 24.955 and 17.671, respectively, according to [23] We analyse the images of the cel1 being pulled into the trap by the optical tweezers with cross-correlation calculation, and obtain the optical trap stiffness by first-order exponential fitting for the displacement of the cell versus time. The optical trap stiffness is determined as ~10 pN μm −1 at the trapping position. Optical tweezers in vivo can be used to study rheology, such as the hemodynamic parameters. The calibration of optical tweezers in vivo is the basis of such applications for quantitative measurements of biological activity. However, some problems need to be solved to use optical tweezers for quantitative measurements in vivo . Among the challenges, we think that the key issue is the reproducibility of optical stiffness calibration. The optical stiffness at different trapping locations varies because of different components within the biological tissue. All the experiments with oil-immersion objectives as here are performed at a depth of ~40 μm. At deeper locations of the mouse ear (>60 μm), optical tweezers have not been able to trap the cells. This can be due to two main reasons: first, the trapping force is reduced significantly by the loss of laser power at a deeper location; second, there might not be an appropriate gradient force to hold the cells, because the level of aberration in focusing through thicker tissue is more severe. Higher laser power and optimization of optical tweezers, such as by wave front correction with a spatial light modulator that has been shown to be efficient to trap through turbid media [25] , could help achieving optical manipulation of cells at deeper locations within living animals. Heat-induced cell damage is a serious problem for investigations involving live animals. When the trapping laser power at the spot in vivo is 168 mW, we do not observe noticeable thermal damage to the trapped cells at the depth of ~40 μm in our experiments. This might have two reasons: first, the trapped cells have good heat conductance (due to water content); second, the trapped cells are immersed in the flowing blood. The blood flow in vivo might also help reducing any possible heat accumulation. Therefore, there is not visible thermal damage by laser light absorption to the trapped cells. Most of the laser power is lost before arriving at the trapping location, because of laser scattering and absorption by the tissues. However, the laser absorption does not damage the tissues in the experiments, because the main component of the biological tissues is water with good heat conductance. In addition, the laser is not focused in the tissues. In our trapping experiments, we do not observe platelets in the images or movies. RBCs are much more common than the other blood cells: there are about 10.4 × 10 6 RBCs, about 0.7 × 10 6 –1.2 × 10 6 platelets and about 1.25 × 10 3 white blood cells in per cubic millimeter of mouse blood [26] . The amounts of all kinds of other cells in capillaries are low due to the slow flow. When the capillaries are blocked, there is no flow passing through the clot, including the platelets. There might be platelets flowing in large vessels. However, the cell images are blurred; thus, the platelets cannot be distinguished. Therefore, platelets are not seen in the images or movies. Previous observations of cellular activity and intercellular interaction in vivo depend on free movement and random pairing of cells, which has low efficiency. Optical trapping has now become an available tool, allowing manipulation of live cells in three dimensions within living animals. It can be used to manipulate targeted cells and orientate them to targeted position, or for intercellular pairing with any orientation. For example, leukocytes can traffic to various tissue compartments under a broad range of physiological and pathological conditions. The infiltration of monocytes is a biological phenomenon in vivo . We believe that using optical trap to fix immune cells to the endothelium may be helpful to study infiltration processes in detail in vivo . In conclusion, we have achieved optical trapping and manipulation of flowing RBCs in blood capillaries of living animals for the first time. The RBCs are trapped in individual blood capillaries. The optical stiffness is also estimated in the paper. In addition, the capillaries are blocked with RBCs trapped by optical tweezers. Furthermore, we have managed to clear the blockage of capillary and recover the blood flow with optical tweezers. These results show great potential of optical tweezers in studying life science in vivo , including processes such as cell migration, cell sorting and targeted drug delivery. Optical tweezers setup Optical tweezers are capable of manipulating micrometre-sized dielectric particles by exerting extremely small forces via a highly focused laser beam. The beam is typically focused by sending it through a microscope objective. In typical optical tweezers, a high numerical aperture objective is used to focus laser beam tightly for three-dimensional potential well. Our optical tweezers setup is based on an Olympus IX71 inverted microscope as shown in Fig. 5a . The microscope is a universal infinity-corrected optical system. A 1,064-nm laser (Amonics, Hong Kong, AFL-1064-37-R-CL) is used as the trapping laser source. This laser beam is expanded by a beam expander to overfill the pupil of microscope objective. Lens L1 ( f =250 mm) focuses the laser beam to the conjugate point of the microscope objective as shown in Fig. 5a after the beam is reflected by mirrors M1 and M2. The laser beam is then directed into the microscope and reflects upward by a dichroic mirror and refocuses into the ear of the mouse after passing through lens L2 (L2 is the tube lens inside the microscope with f =180 mm) and a microscope objective (oil immersion, × 100, numerical aperture=1.25, Jiangnan, China). The images are recorded by a CCD (Coolsnap cf, USA, 7 frames per second), and acquired by Image-Pro Express (IPE) movie capture software. 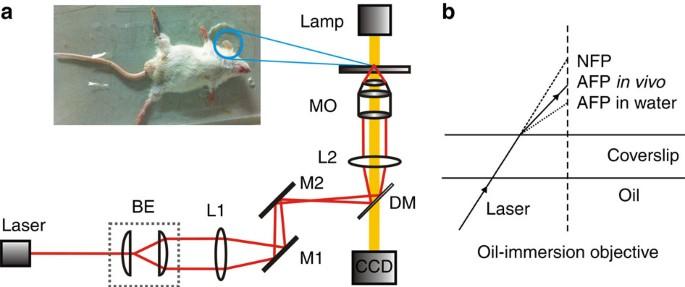Figure 5: Optical tweezers setup. (a) Instrument layout showing optical paths for 1,064 nm trapping laser (red) and halogen lamp for bright-field imaging (yellow). BE, beam expander; L1–L2, lens; M1–M2, mirrors; MO, microscope objective; DM, dichroic mirror. The inset shows the ear of the mouse at the sample stage. (b) The geometric optics representation of the refraction of a light beam focusedin vivo. NFP, nominal focal position; AFP, the actual focal position. Figure 5: Optical tweezers setup. ( a ) Instrument layout showing optical paths for 1,064 nm trapping laser (red) and halogen lamp for bright-field imaging (yellow). BE, beam expander; L1–L2, lens; M1–M2, mirrors; MO, microscope objective; DM, dichroic mirror. The inset shows the ear of the mouse at the sample stage. ( b ) The geometric optics representation of the refraction of a light beam focused in vivo . NFP, nominal focal position; AFP, the actual focal position. Full size image Usually, optical trapping force decreases dramatically with the increase of trapping depth, owing to spherical aberration, which is induced by a mismatch in the refractive indices of the specimen and the immersion oil [27] . The aberrations of trapping laser beam in vivo and in water are shown in Fig. 5b , respectively. Typical refractive index of skin tissue is about 1.4 ( [28] ), which is larger than the refractive index of water (1.33). The difference of refractive indices leads to different spherical aberrations of optical trapping in vivo and in water. The actual focus position in vivo is closer to the nominal focal position compared with the actual focal position in water. The reduction in spherical aberration by using an oil-immersion objective is helpful for trapping cells in vivo . The investigation reported by Reihani et al . [29] has shown that the aberration induced by the mismatch of refractive indices can be balanced by changing the tube length, which leads to a shift in the position of the maximum trapping force in the longitudinal direction. Such spherical aberration compensation technology is used in the building of our current optical tweezers for in vivo trapping. The microscope objective used in our experiments is in standard finite-tube length (160 mm) mode. The laser beam is a parallel light before entering the objective. According to previous results, the maximum trapping efficiency of optical tweezers occurs at the depth of ~50 μm [30] . Animals BALB/c mice (6-week-old, 20±2 g) were purchased from the Experimental Animal Center of Anhui Medical University and were anaesthetized with 20% urethane (1.0 g kg −1 ) via injection to hip muscles. The hair of mice was removed at the ear skin by a razor after anaesthetization. The mouse ear was then carefully put on a coverslip with glycerin for microscopy observation as shown in the inset of Fig. 5a . The glycerol layer was about 10 μm thick. RBCs were at the depth of ~40 μm beneath the surface of mouse ear skin. Therefore, the trapping depth in the experiments was ~50 μm. The study was approved by the Ethical Committee of the University of Science and Technology of China. Estimation of focal laser power We measure the focal laser power with dual-objective technology [31] . There is immersion oil between the objective lens and sample to collect laser light as much as possible. Two coverslides are used to fix the tissue slices. The laser power after the tissue slices is measured to estimate the focal laser power in vivo . The laser power is measured as 404 mW before entering the biological tissues. We use three slices for measurements with each slice measured at five different locations. From the measurement results, we estimate that the focal laser power in vivo is about 168 mW (biological tissue: mouse ear; slice thickness: 40 μm; equipment: Leica CM 1950 Microsystems, Germany). How to cite this article : Zhong, M.-C. et al . Trapping red blood cells in living animals using optical tweezers. Nat. Commun. 4:1768 doi: 10.1038/ncomms2786 (2013).